Hydrogen-atom-mediated electrochemistry Silicon dioxide thin films are widely used as dielectric layers in microelectronics and can also be engineered on silicon wafers. It seems counterintuitive that electrochemical reactions could occur on such an insulator without relying on tunnelling current. Here we report electrochemistry based on electron transfer through a thin insulating layer of thermally grown silicon dioxide on highly n-doped silicon. Under a negative electrical bias, protons in the silicon dioxide layer were reduced to hydrogen atoms, which served as electron mediators for electrochemical reduction. Palladium nanoparticles were preferentially formed on the dielectric layer and enabled another hydrogen-atom-mediated electrochemistry, as their surfaces retained many electrogenerated hydrogen atoms to act as a ‘hydrogen-atom reservoir’ for subsequent electrochemical reduction. By harnessing the precisely controlled electrochemical generation of hydrogen atoms, palladium–copper nanocrystals were synthesized without any surfactant or stabilizer on the silicon dioxide layer. Precise control of electrochemical reactions on dielectric layers is a key issue that has been increasingly studied in recent years, because it would enable patterned circuits, stacks of thin films and various nanoparticles (NPs) to be fabricated on dielectric layers by direct electroplating. Although electrochemistry on dielectric layers has the potential to offer new fundamental methodologies in various fields such as the semiconductor industry, energy conversion, sensors, catalysts and supercapacitors, there have been relatively few studies on this topic, mainly because it is counterintuitive that electrochemical reactions could occur on dielectric layers, that is, insulators. In fact, electrochemistry through insulators such as glass [1] , metal oxide [2] , [3] , organic monolayers [4] and rubbed Teflon [5] has been investigated. Previous studies have reported on electrochemistry through amorphous glass films [1] , which have many pores that permit the penetration of redox species and ions. Because of the permeability of many chemical species, no electron mediator was required to be in the glass membrane for a faradaic reaction. A silicon (Si) electrode modified with an organic monolayer is another example that has been intensively investigated over the past decades. The reproducible fabrication of stable and sufficiently thick dielectric layers has been found to be crucial for informative and practical systems. Silver (Ag) NPs were electrodeposited on aluminum (Al) oxide at −9 V (ref. 3 ) and the direct electrochemical reduction [2] of TiO 2 to Ti was performed at 950 °C. Rubbed Teflon was also adopted as an insulator on which metal was deposited [5] . Although such studies have suggested new approaches to introducing electrochemistry to insulating materials (dielectrics), there are still challenges to adapting these approaches to practical applications, including the permeability, reproducibility, temperature and controllability of the electrochemical reaction. More importantly, only a limited number of studies have investigated electrochemistry processes that occur at the dielectric layer. In this work, we introduced thermally grown silicon dioxide (SiO 2 ), a dense and stable dielectric layer, and explored the novel phenomena that could be observed in this electrochemical system. Thermal SiO 2 is a dielectric material used for conventional metal/insulator/metal capacitors [6] , and SiO 2 films are widely used as gate insulators of metal/oxide/semiconductor (MOS) devices [7] , in which the field-induced drift of protons to the Si/SiO 2 interface and their interactions with electrons can create hydrogen (H) atoms at the interface [8] , [9] . Shkrob et al. [10] demonstrated that protons were reduced to generate mobile H atoms in B 2 O 3 glasses at room temperature. Energy calculations revealed that H atoms in SiO 2 are isolated by themselves without a strong interaction with oxygen (O 2 ) or Si atoms. H atoms reside in interstitial sites ~2.0 Å away from the nearest O 2 atoms and do not disturb the surrounding lattice [11] . Schrauben et al. [12] provided evidence for H atom transfer through reduced TiO 2 and ZnO NPs in solution using two H abstractors, namely, 2,4,6-tri-tert-butylphenoxyl radical ( t Bu 3 ArO·) and 2,2,6,6-tetramethyl-piperidin-1-yl-oxyl. Revesz [13] studied on an electrolyte/oxide/Si (EOS) system to determine the concentration of certain active H-bearing species in the oxide. The highly n-doped Si/thermal SiO 2 thin layers in an aqueous electrolyte considered in this work represent an EOS system suitable for producing H atoms electrochemically by finely tuning the applied potential bias and pH of the solution. The SiO 2 thin film, which is thermally grown on highly n-doped Si (the fabrication method and properties are described in detail in Methods and the Supplementary Information ), has a highly dielectric structure with minimal defects. Therefore, it permits both the selective migration of protons and the diffusion of electrogenerated H atoms [9] in the middle of the electrical potential gradient. This result suggests that H atoms in the EOS system could be used as electron mediators on dielectric oxide layers acting as ‘chemical electrodes’ for electrochemical reactions. Free H atoms are theoretically very strong reducing agents (−2.106 V versus normal hydrogen electrode) [14] . In the proposed system of highly n-doped Si/thermal SiO 2 thin layers, the reducing power of H atoms in SiO 2 should not be as strong as that of freestanding H atoms. However, the well-ordered SiO 2 structure provides a remarkably stable and inert environment. H atoms in titanium dioxide (TiO 2 ) and zinc oxide (ZnO) are strongly bound and act as a dopant but weakly interact with the neighbouring oxygen atoms in SiO 2 (refs 10 , 15 ). Thermally grown SiO 2 is not expected to modify the chemical properties of the interstitial H atoms to the same degree as TiO 2 (ref. 11 ) and ZnO (ref. 16 ). Therefore, in the proposed system, electrogenerated H atoms would serve as sufficiently strong reducing agents to reduce most reducible species in solution. Next, metal precursors could be electroplated by H atoms on the thermal SiO 2 surface to potentially form the corresponding metal NPs. This process could offer important inspiration for many interesting applications in that various metal NPs adsorbed on oxide surfaces are widely used for energy technology, pollution prevention and environmental clean-up efforts [17] , [18] . In particular, SiO 2 is commonly used as an inert support for heterogeneous catalysts. Compared with chemical reduction, electrochemical methods enable fine and easy control by electronic devices and primarily require no reducing agents because of the direct injection of electrons [19] . Therefore, electroplating has been considered as an alternative method for the cost-effective and stabilizer-free NP preparation. However, long-term electrochemical operation requires appropriate electrodes that must be safely free from passivation to continue providing electrons for sustainable faradaic reactions. Many electrodes are subject to deactivation, which is mostly caused by the irreversible adsorption of adsorptive intermediates and/or the deterioration of electrode materials by reactive species. Herein, we report electron transfer through a thin insulating layer of the 6-nm-thick thermal SiO 2 on highly n-doped silicon (n + -Si), leading to unprecedented electrochemistry on the dielectric surface. Under a negative electrical bias, protons from the solution media migrate into the silicon dioxide layer and produce significant cathodic current. The asymmetric voltammograms from the proposed system suggest electrogeneration of H atoms as electron mediators for electrochemical reduction at the interface between the dielectric surface and solution. By precisely tuning the voltammetric conditions, palladium (Pd)–copper (Cu) nanocrystals (NCs) are synthesized without any surfactant or stabilizer, and both O 2 and carbon dioxide (CO 2 ) are electrochemically reduced on the SiO 2 layer. SiO 2 layers in the EOS system The thermally grown SiO 2 considered in this work has an exact stoichiometric composition [20] . Supplementary Fig. S1 presents high-resolution transmission electron microscopy (HRTEM) cross-sectional images of the high n + -Si/SiO 2 (6-nm thick). A compact SiO 2 layer was uniformly formed on Si; this layer was very stable as demonstrated by the tests of breakdown voltage and metal electroplating ( Supplementary Figs S2 and S3 ; Supplementary Note 1 ). The n + -Si/SiO 2 immersed in an aqueous solution was used as the working electrode to investigate the electrochemistry in this system, as illustrated in Fig. 1 . The linear sweep voltammogram ( i – V curve) obtained in the proposed EOS system using the n + -Si/SiO 2 electrode demonstrates that the 6-nm-thick thermal SiO 2 clearly differed from the native SiO x on n + -Si ( Supplementary Fig. S4 ). Compared with the native SiO x layer, the structure of the thermal SiO 2 is sufficiently dense and uniform for the background current to be negligible, providing a reliable system for electrochemical study. 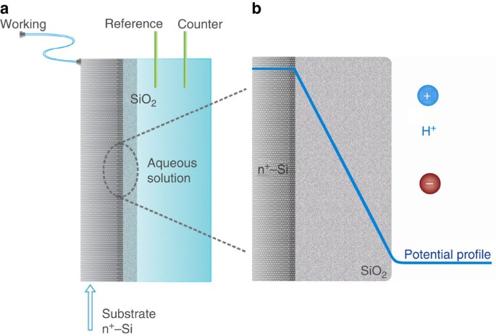Figure 1: Schematic view of the electrochemical experiment. (a) Experimental system and (b) schematic representation of the electrical potential profile across highly n-doped Si (n+-Si)/thermal SiO2/aqueous electrolyte. Figure 1: Schematic view of the electrochemical experiment. ( a ) Experimental system and ( b ) schematic representation of the electrical potential profile across highly n-doped Si (n + -Si)/thermal SiO 2 /aqueous electrolyte. Full size image In previous studies, the electrical potential distribution across the Si/SiO 2 interface in an EOS system was not significantly different from that in a MOS system [21] . In contrast to the solution in an MOS configuration, the solution in an EOS system acts as an infinite source of ions that can be polarized near the oxide surface upon the application of an electric field as long as the dielectric layer is sufficiently thin to incompletely isolate the conducting Si phase from the solution, in electrical terms [7] . However, the applied electrical potential still drops mainly across the oxide layer because of its high resistance of 10 7 Ω cm 2 , for the thermally grown 6-nm-thick SiO 2 layer on n + -Si, as measured by impedance analysis ( Supplementary Note 2 ). The electrical potential drop at the 6-nm-thick SiO 2 layer was 2 × 10 5 times greater than that at the SiO 2 /solution interface in this EOS system ( Supplementary Fig. S5 ). Therefore, the potential difference at the interface between SiO 2 and the solution is negligible compared with the entire applied bias. 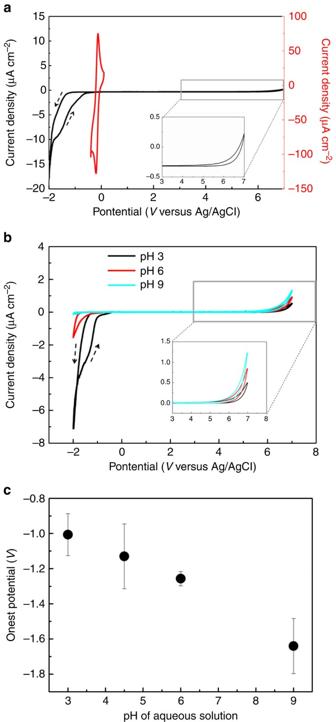Figure 2: Electrochemistry of the proposed EOS system. (a) Cyclic voltammograms (CVs) of the n+-Si/SiO2electrode (black) and GC electrode (red) were recorded at room temperature in an N2-purged solution of 1 mM Ru(NH3)6Cl3+Ru(NH3)6Cl2+0.1 M potassium phosphate solution at pH 3 with a scan rate of 10 mV s−1. (b) CV curves of the n+-Si/SiO2(6-nm thick) electrode were obtained in 0.1 M phosphate buffer at pH 3 (black), pH 6 (red) and pH 9 (bright blue). The insets inaandbpresent the enlarged portion of the CV for the anodic potential at the n+-Si/SiO2electrode. (c) The onset potential depending on the pH inb. The onset potential was determined at the potential at which the current density is above 30% compared with the baselines. The voltammograms were obtained at 10 mV s−1at room temperature under N2. Electron transfer through the SiO 2 dielectric layer Figure 2a presents the cyclic voltammograms recorded using an n + -Si/SiO 2 electrode and the comparison of these voltammograms with that obtained using a glassy carbon (GC) electrode, in 0.1 M potassium phosphate buffer solution at pH 3. The electrochemical oxidation of Ru(NH 3 ) 6 2+ at the n + -Si/SiO 2 required a considerably higher overpotential than the GC electrode. The onset potential was observed at approximately +3.2 V (versus Ag/AgCl), and the current increased gradually as the potential increased in the positive direction. In contrast, the overpotential for Ru(NH 3 ) 6 3+ reduction was far lower than expected from the oxidation results in the same system. The faradaic current for reduction sensitively responded to the electrical potential bias, despite the compact dielectric layer of thermally grown SiO 2 . In addition, Fig. 2b,c demonstrates that the onset potential of an n + -Si/SiO 2 electrode systematically depended on the pH of the aqueous electrolyte in the cathodic regime, whereas no pH dependence was observed in the anodic region. The asymmetric voltammogram in Fig. 2a strongly implies that there are electrochemically reducible species inside the SiO 2 layer, preferentially taking up electrons from the highly doped Si phase. Figure 2: Electrochemistry of the proposed EOS system. ( a ) Cyclic voltammograms (CVs) of the n + -Si/SiO 2 electrode (black) and GC electrode (red) were recorded at room temperature in an N 2 -purged solution of 1 mM Ru(NH 3 ) 6 Cl 3 +Ru(NH 3 ) 6 Cl 2 +0.1 M potassium phosphate solution at pH 3 with a scan rate of 10 mV s −1 . ( b ) CV curves of the n + -Si/SiO 2 (6-nm thick) electrode were obtained in 0.1 M phosphate buffer at pH 3 (black), pH 6 (red) and pH 9 (bright blue). The insets in a and b present the enlarged portion of the CV for the anodic potential at the n + -Si/SiO 2 electrode. ( c ) The onset potential depending on the pH in b . The onset potential was determined at the potential at which the current density is above 30% compared with the baselines. The voltammograms were obtained at 10 mV s −1 at room temperature under N 2 . Full size image These electrochemically reducible species can be identified from the following process. First, the cathodic onset potential of the n + -Si/SiO 2 electrode in an aprotic organic electrolyte, such as acetonitrile, was observed at approximately −2.2 V (versus Ag/Ag + ; Supplementary Fig. S6 ). The cathodic current disappeared without a proton. Second, the behaviour in acetonitrile follows the Fowler–Nordheim tunnelling ( Supplementary Fig. S7 ), which is similar to MOS systems [22] . When a small amount of proton sources, HClO 4 , was added to the solution, the cathodic current began to flow at a more positive value of approximately −1.2 V, whereas the background current was negligible in the same potential range ( Supplementary Fig. S8 ). The proton sources clearly caused the system to deviate from the Fowler–Nordheim tunnelling model ( Supplementary Note 3 ), revealing that the proposed system cannot be explained by a simple direct tunnelling model. Third, the thermal SiO 2 layer in this system completely blocks permeation of all chemical species, including Ru(NH 3 ) 6 2+/3+ ions and electrolytes, except protons, which can diffuse through the SiO 2 interfacial plane [23] and reversibly migrate back and forth in response to an external electric field [24] . This evidence unequivocally supports the conclusion that the cathodic currents in the linear sweep voltammograms in Fig. 2 were attributed to protons, which can migrate into the SiO 2 layer and be electrochemically reduced ( Supplementary Note 4 ). Figure 2a reveals that the current in the forward scan in the negative potential region was smaller than that in the reverse scan. This result again demonstrates that the thermal SiO 2 layer in the proposed system is not a simple insulator through which a tunnelling current predominantly flows. During the period in which a negative potential was applied, protons accumulated in the SiO 2 layer and were electrochemically reduced to H atoms. This result is ensured by a comparison of the consecutive scans in linear sweep voltammetry. The onset potential of the second scan, which was performed immediately after the first scan, shifted in the positive direction and the cathodic current increased ( Supplementary Fig. S9 ). The H atoms remaining inside the SiO 2 layer, which were generated during the previous scan, could relay electrons to the protons originating from the solution via homogeneous electron exchange. The onset potential was restored after leaving the electrode in a solution for ~1 h without any electrical bias ( Supplementary Fig. S9 ). 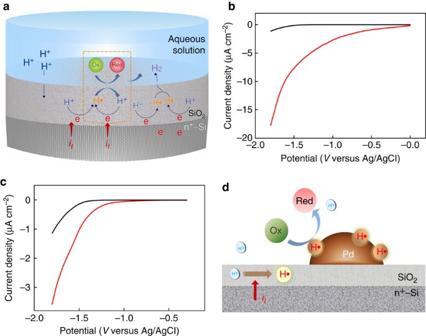Figure 3: CO2and O2reduction and Pd NPs acting as H-atom lagoons. (a) Schematic view of the reactions in the proposed system: H-atom-mediated electron transfer in n+-Si/thermally oxidized SiO2/aqueous solution. Protons in the aqueous solution drift into the SiO2layer and become H atoms by capturing electrons tunnelling through the Si/SiO2interface under a negative potential. (b) The linear sweep voltammogram of n+-Si/thermally oxidized SiO2in black was obtained at room temperature in an N2-purged solution of 0.1 M potassium phosphate at pH 3. The linear sweep voltammogram in red was obtained at room temperature in a CO2-saturated solution of 0.1 M potassium phosphate at pH 3. (c) The linear sweep voltammogram of n+-Si/thermally oxidized SiO2in black was obtained at room temperature in an N2-purged solution of 0.1 M potassium phosphate at pH 3. The linear sweep voltammogram in red was obtained at room temperature in an O2-saturated solution of 0.1 M potassium phosphate at pH 3. (d) Schematic illustration of the H-atom lagoon effect of Pd NPs on n+-Si/SiO2(thermally oxidized) for the reduction of reducible species. Figure 3a illustrates how the migration and reduction of protons in the SiO 2 layer can enable the reduction of redox species without a direct tunnelling current despite the presence of the dense insulating SiO 2 layer. The electrogenerated H atoms either directly serve as electron mediators or form H 2 molecules at the SiO 2 /solution interface. Figure 3: CO 2 and O 2 reduction and Pd NPs acting as H-atom lagoons. ( a ) Schematic view of the reactions in the proposed system: H-atom-mediated electron transfer in n + -Si/thermally oxidized SiO 2 /aqueous solution. Protons in the aqueous solution drift into the SiO 2 layer and become H atoms by capturing electrons tunnelling through the Si/SiO 2 interface under a negative potential. ( b ) The linear sweep voltammogram of n + -Si/thermally oxidized SiO 2 in black was obtained at room temperature in an N 2 -purged solution of 0.1 M potassium phosphate at pH 3. The linear sweep voltammogram in red was obtained at room temperature in a CO 2 -saturated solution of 0.1 M potassium phosphate at pH 3. ( c ) The linear sweep voltammogram of n + -Si/thermally oxidized SiO 2 in black was obtained at room temperature in an N 2 -purged solution of 0.1 M potassium phosphate at pH 3. The linear sweep voltammogram in red was obtained at room temperature in an O 2 -saturated solution of 0.1 M potassium phosphate at pH 3. ( d ) Schematic illustration of the H-atom lagoon effect of Pd NPs on n + -Si/SiO 2 (thermally oxidized) for the reduction of reducible species. Full size image Electrochemical reduction of CO 2 and O 2 in the EOS system The H-atom-mediated electrochemistry of this simple n + -Si/SiO 2 /aqueous electrolyte system could be used for the electrochemical reduction of CO 2 and O 2 , which involves strongly reactive or adsorptive intermediates. In particular, the reductive transformation of CO 2 to fuels and commodity chemicals is one of the most important contemporary energy and environmental challenges. The initial step from CO 2 to CO 2 ·− has been reported to be rate limiting in many cases. Either the overpotentials are exceedingly high or the metal surface becomes deactivated by the intermediates [25] , [26] . The long-term stability of the electrodes is a crucial challenge in making electrochemical CO 2 reduction economically feasible [26] . Figure 3b demonstrates the CO 2 reduction in this system. The product of CO 2 reduction in this system was mainly formic acid at −1.5 V (versus Ag/AgCl) in CO 2 -saturated aqueous solution at pH 3 for longer than 4 h. H atoms that were not used for CO 2 reduction are expected to form molecular hydrogen. Both O 2 and CO 2 can be reduced in this system ( Fig. 3c ) without significant deterioration of the oxide structure by electrolysis over 1 h. Bimetallic NCs synthesized electrochemically on the SiO 2 layer The finely controllable H-atom-mediated electrochemistry of the n + -Si/SiO 2 (6-nm thick)/aqueous electrolyte system was used for the electrodeposition of several types of metals. Direct electron tunnelling can reduce metal precursors on native silicon oxide, producing 1- to 2-nm-thick non-adherent powders that are readily washed off by rinsing [27] . In contrast, the Pd NPs (diameter of 10–40 nm) formed in this system were uniformly distributed on the oxide layer due to the reduction of Pd 2+ ions to metallic Pd ( Supplementary Fig. S10 ). The Pd NPs were anchored so strongly that very few were washed off by rinsing. H 2 molecules are likely to prevent the initial Pd seeds from aggregating, resulting in immobilization [28] , and thus, H atoms, which are much stronger reducing agents, are assumed to have a pivotal role in the prompt reduction of Pd 2+ ions. Thus, this system enables the single-step electrochemical fabrication of Pd NPs firmly adhered to the SiO 2 layer in aqueous solution at room temperature without surfactants or stabilizers. Pd NPs prepared in this manner are expected to have application in hydrogen storage as catalysts on solid supports and as sensing devices [29] . Metallic Pd is well known to retain H atoms on its surface. Once Pd NPs are formed on the SiO 2 layer, the excess H atoms are predicted to be adsorbed on the surfaces of the Pd NPs spontaneously at room temperature. Even if H 2 molecules are formed, they would be readily dissociated on the Pd surface [29] . Thus, the hydrogen-rich surfaces of the Pd NPs are expected to facilitate deposition of metals, such as Cu, which otherwise do not adhere to the SiO 2 surface [27] . The Pd NPs on the SiO 2 surface in this system act as ‘H-atom lagoons’ that collect and store as many H atoms as they can on their surfaces, as demonstrated in Fig. 3d . Such a novel H-atom lagoon leads to the subsequent electroplating of various metals, including bimetallic NCs. Bimetallic NCs are of considerable interest because of their unique properties and potential applications [30] , [31] . H-atom-mediated electrochemistry employing H-atom lagoons, such as those formed by Pd NPs on SiO 2 , can achieve facile bimetallic NC synthesis with a polyhedral alloy on an inert support. 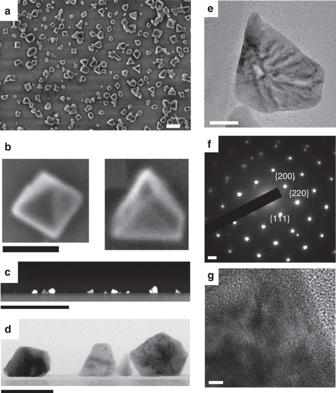Figure 4: Pd–Cu NCs. (a) FESEM image of Pd–Cu NCs prepared as follows. First, a constant potential of −1.2 V was applied to n+-Si/SiO2for 30 min in 1 mM PdCl2+0.1 M potassium phosphate solution at pH 3. Next, SiO2-supported Pd NPs were immersed in 1 mM CuSO4+0.1 M H2SO4solution and a constant potential of −1.3 V was applied for 30 min. Scale bar, 200 nm. (b) High-magnification FESEM image of Pd–Cu NCs prepared as ina. Octahedron-shaped Pd–Cu NCs (left), triangular-prism-shaped Pd–Cu NCs (right). Scale bar, 100 nm. (c) High-angle annular dark field-scanning TEM image of SiO2-supported Pd–Cu NCs prepared as ina. Scale bar, 1 μm. (d) TEM image of Pd–Cu NCs. Scale bar, 100 nm. (e) TEM image of Pd–Cu NCs. Scale bar, 20 nm. (f) Electron diffraction pattern of NCs. Scale bar, 2 nm−1. (g) HRTEM image of a single Pd–Cu NC. Scale bar, 2 nm. Figure 4a presents electron microscopic images of polyhedral Pd–Cu bimetallic NCs consisting of octahedron (32%), triangular prisms (38%) and others (30%). This study represents the first electrochemical shape-controlled synthesis of bimetallic NCs without any stabilizer or surfactant. Energy-dispersive spectroscopy (EDS) revealed that the electroplated Pd–Cu bimetallic NCs were a Pd–Cu mixed alloy ( Supplementary Fig. S11 ). The TEM image and corresponding electron diffraction pattern of a single Pd–Cu NC in Fig. 4f indicate that the NC was a piece of a single crystal enclosed by {111}, {200} and {220} facets. In addition to Pd–Cu NCs, Pd–Au NCs and Pd–Co NCs were also synthesized on a thin SiO 2 layer at room temperature without the aid of a stabilizer or additive ( Supplementary Figs S12 and S13 ). Figure 4: Pd–Cu NCs. ( a ) FESEM image of Pd–Cu NCs prepared as follows. First, a constant potential of −1.2 V was applied to n + -Si/SiO 2 for 30 min in 1 mM PdCl 2 +0.1 M potassium phosphate solution at pH 3. Next, SiO 2 -supported Pd NPs were immersed in 1 mM CuSO 4 +0.1 M H 2 SO 4 solution and a constant potential of −1.3 V was applied for 30 min. Scale bar, 200 nm. ( b ) High-magnification FESEM image of Pd–Cu NCs prepared as in a . Octahedron-shaped Pd–Cu NCs (left), triangular-prism-shaped Pd–Cu NCs (right). Scale bar, 100 nm. ( c ) High-angle annular dark field-scanning TEM image of SiO 2 -supported Pd–Cu NCs prepared as in a . Scale bar, 1 μm. ( d ) TEM image of Pd–Cu NCs. Scale bar, 100 nm. ( e ) TEM image of Pd–Cu NCs. Scale bar, 20 nm. ( f ) Electron diffraction pattern of NCs. Scale bar, 2 nm −1 . ( g ) HRTEM image of a single Pd–Cu NC. Scale bar, 2 nm. Full size image The remarkably low onset potential ( Fig. 2a ) for the cathodic reaction indicates that protons were reduced inside the SiO 2 layer. Thus, the observed voltammetric results can be understood by a scenario in which an external electric field causes protons to migrate in the oxide layer [24] and the protons are electrochemically reduced to produce H atoms [9] , [32] in a negative potential regime. Shkrob et al. [10] suggested that electrons react with network-bound protons at 180–530 K to produce H atoms. We applied a negative potential to an n + -Si/SiO 2 electrode in 0.1 M potassium phosphate buffer solution at pH 3 and acquired surface-enhanced Raman scattering (SERS) spectra from the SiO 2 layer. The peak of the Si–(OH + )–Si complex [33] at ~2,905 cm −1 was observed ( Supplementary Fig. S14 ) in accordance with the suggested mechanism [10] . This observation confirms the permeation of protons into the SiO 2 layer and supports the idea that H atoms can be generated because of proton reduction in the SiO 2 layer under an external electric field. The presence and role of H atoms as electron mediators in the SiO 2 layer can be verified by independent voltammetric experiments using several redox-active species with different reduction potentials. Although redox-active species are characteristically reduced at different potentials on conventional conducting electrodes, such as GC and Au, their reduction behaviour in this system exhibited no correlation with the reduction potentials of their own (not shown). This result cannot be explained by a direct tunnelling current. The electrochemical reduction of iridium (Ir) precursors ( Supplementary Fig. S15 ) provides additional evidence of the electrogeneration of H atoms in the SiO 2 layer. Although the Ir precursors used in this study require a very negative potential or commensurately strong reducing agent to be reduced, metallic Ir NPs were electrodeposited on the SiO 2 surface at a moderate potential bias of −1.3 V. Considering the monotonously linear and predominant drop of electrical potential across the SiO 2 film ( Fig. 1 ), it is unlikely that a direct tunnelling current is responsible for this result. The experiment indicated that the Ir precursors are not reduced by H 2 molecules but may be reduced by H atoms [34] , [35] . In this study, we propose and investigate H-atom-mediated electrochemistry in the system of n + -Si/thermal SiO 2 /aqueous solution in which a thin and dense SiO 2 layer acted as a proton-selective membrane and reservoir of atomic H. In voltammetry, the redox current was not linearly dependent on the external potential bias, and reduction occurred at a lower overpotential in proton-rich solutions compared with oxidation, resulting in asymmetric voltammetric behaviour. The experimental evidences unequivocally demonstrates that protons from the solution permeated into the SiO 2 layer and were reduced to form H atoms by the uptake of electrons from the highly doped Si phase under a negative potential. The electrogenerated H atoms diffuse into the SiO 2 layer and reduce the precursors, having the role of electron mediators. The suggested mechanism is in good agreement with the observed nonlinear and asymmetric voltammetric behaviour. The proposed H-atom-mediated electrochemistry can be used to synthesize Pd NPs with an average size of 10–30 nm without using stabilizers or additives ( Supplementary Fig. S10 ). More importantly, the Pd NPs on the SiO 2 layer can act as a H-atom lagoon for the facile nanofabrication of bimetallic NCs such as Pd–Cu, Pd–Au and Pd–Co. In particular, the system in this study successfully demonstrated its potential for producing various metallic nanostructures, including Pd–Cu bimetallic NCs, with such shapes as triangular prisms and octahedron on the SiO 2 substrate. Both bimetallic NCs and monometallic NPs were synthesized on the SiO 2 in the absence of any additive or stabilizer. H-atom-mediated electrochemistry will provide an impetus to the future fabrication of electronic circuits, sensory units and thin-film-based energy conversion devices on insulating layers. Preparation of thermal oxidized SiO 2 N-type (n + -Si), phosphorous-doped, <100> oriented Si wafers with a resistivity as low as 0.005 Ω cm were obtained from STC (Japan). Highly n-doped Si with thermally oxidized SiO 2 (n + -Si/SiO 2 ) was prepared via conventional thermal oxidation of highly doped Si wafers (<100>, n-type, 0.005 Ω cm). After cleaning with a mixture of H 2 SO 4 and H 2 O 2 , the native oxide was stripped by HF dipping and the 200-Å-thick thermal oxide was produced at 850 °C in a furnace with dry O 2 blowing. Next, 200-Å-thick thermal oxides were stripped again by HF dipping. Cleaning was repeated and the target 50- or 60-Å-thick thermal SiO 2 layer was formed at 850 °C in a furnace with dry O 2 blowing. The thermal SiO 2 layers produced were uniformly flat. Ellipsometry and HRTEM ( Supplementary Fig. S1 ) confirmed that the thicknesses of the thermal SiO 2 layer on Si was 60 Å. Chemicals and electrochemical experiments Before every experiment, the samples were degreased by sonication in acetone and isopropanol, and rinsed with methanol or deionized water. For back contact, the back side of the wafer sample was scratched with a diamond knife to remove the air-formed SiO 2 film followed by smearing with a Ga–In eutectic. This surface was then pressed to a metal support. The ohmic nature of the contact was verified by electrical measurements. After this procedure, the samples were pressed against the O-ring of an electrochemical cell, leaving 0.066 cm 2 exposed to an aqueous solution of 0.1 M potassium phosphate (Daejung Chemicals & Metals Co., Ltd) in deionized water. A pH electrode (ROSS 8102, Orion) was used to adjust the pH of the aqueous solution for electrochemical measurement. The electrochemical experiments were performed at room temperature in a three-electrode electrochemical cell connected to a potentiostat (750, CHI Instruments, Inc.). An Ag/AgCl (in 3 M NaCl, BAS Inc.) and Pt wire (diameter 0.5 mm) were used as reference and counter electrodes, respectively. Cyclic voltammograms and linear sweep voltammograms were obtained with or without redox species after purging with N 2 for 20 min. Hexaammineruthenium(II) chloride (Ru(NH 3 ) 6 Cl 2 , ≥99.9% trace metal basis), hexaammineruthenium(III) chloride (Ru(NH 3 ) 6 Cl 3 , 98%) and Ir (III) chloride hydrate (Ir 3 Cl·xH 2 O, ≥99.9% trace metal basis) were purchased from Sigma-Aldrich for use as redox species. For CO 2 and O 2 reduction, Si (n + -Si)/SiO 2 (6-nm thick) was used as a working electrode; this electrode was exposed to 0.1 M potassium phosphate buffer at pH 3 after rinsing with deionized water. The aqueous solution was purged with CO 2 or O 2 gas for at least 20 min. An Ag/AgCl (in 3 M NaCl, BAS, Inc.) and Pt mesh were used as reference and counter electrodes, respectively. For CO 2 reduction, after applying a constant potential of −1.5 V (versus Ag/AgCl) to the working electrode for 4–8 h, the solution was analysed using HPLC (Dionex, USA) at the National Instrumentation Center for Environmental Management of Seoul National University. SERS on n + -Si/SiO 2 in the EOS system The 11-mercaptoundecanol-modified gold microshell was used for SERS monitoring [36] . The Raman spectra were obtained using a homemade Ramboss Micro-Raman system spectrometer with a TE cooled (−60 °C) charged-coupled device camera (1,024 × 128 pixels). The 632.8 nm line from a He–Ne laser (LASOS Lasertechnik GmbH, USA) was employed as an excitation source and focused through a × 50 objective for in situ electrochemical SERS experiments. The grating (1,200 and 1,800 grooves mm −1 ) and slit provided a spectral resolution of 4 cm −1 . The spectrometer was calibrated with the Raman bands of a silicon wafer at 520 cm −1 and indene at 730.4, 1,018.3, 1,205.6, 1,552.7 and 1,610.2 cm −1 . Ir deposition catalysed by H atoms present on the SiO 2 surface The n + -Si/SiO 2 (6-nm thick) electrode was immersed in an N 2 -purged solution of iridium (III) chloride hydrate and a constant potential of −1.3 V was applied to the electrode. The presence of Ir particles on n + -Si/SiO 2 was confirmed by field-emission scanning electron microscopy (FESEM) and X-ray photoelectron spectroscopy. Supplementary Fig. S11 presents the deposition of Ir, and X-ray photoelectron spectroscopy provided data characteristic of metallic Ir, namely Ir 4f 7/2 and Ir 4f 5/2 peaks at 61.0 and 63.9 eV, respectively. Formation of NCs or NPs on SiO 2 Palladium (II) chloride (PdCl 2 , ≥99.9%), potassium gold (III) chloride (KAuCl 4 , 98%) and cobalt sulfate hydrate (CoSO 4 · × H 2 O, ≥99.9% trace metal basis) were purchased from Sigma-Aldrich. Copper sulphate (CuSO 4 ) was purchased from Junsei Chemicals Co., Ltd. Deposition of Pd NPs on n + -Si/SiO 2 (6-nm thick) was performed in a conventional three-electrode cell with an Ag/AgCl electrode (3 M NaCl, BAS Inc.) and Pt wire (diameter of 0.5 mm) as the reference and counter electrodes, respectively. All potentials refer to the Ag/AgCl reference electrode. The NPs and NCs were electrochemically synthesized in 0.1 M potassium phosphate buffer at pH 3 in an N 2 environment immediately after purging the solution with N 2 gas for 20 min at room temperature. To deposit Pd NPs on the SiO 2 surface, an aqueous solution composed of 0.2–1 mM PdCl 2 in 0.1 M potassium phosphate buffer at pH 3 was prepared and a constant potential of −1.2 V or −1.5 V (versus Ag/AgCl) was applied to the n + -Si/SiO 2 . After Pd deposition on the SiO 2 surface, other metals, including Cu, Au and Co, were deposited on n + -Si/SiO 2 -supported Pd NP electrodes to determine whether Pd-based bimetallic fabrication occurred. For Pd–Cu bimetallic NCs, a 1 mM CuSO 4 aqueous solution in 0.1 M potassium phosphate buffer at pH 3 was prepared and the constant potential of −1.3 V (versus Ag/AgCl) was applied to the n + -Si/SiO 2 -supported Pd NPs electrode. For Pd–Au bimetallic NPs, a constant potential of −1.3 V (versus Ag/AgCl) was applied to the n + -Si/SiO 2 -supported Pd NPs electrode in an aqueous solution of 1 mM KAuCl 4 in 0.1 M potassium phosphate buffer at pH 3. Pd–Co bimetallic NPs were synthesized under −1.8 V (versus Ag/AgCl) applied to the n + -Si/SiO 2 -supported Pd NPs electrode for 30 min. Characterization of NCs and NPs on SiO 2 The NCs and NPs on SiO 2 prepared in the manner described above were characterized by FESEM (Carl Zeiss, Germany) and EDS (Carl Zeiss, Germany) at the National Instrumentation Center for Environmental Management of Seoul National University. For high-resolution images, HRTEM (JEOL, Japan) and EDS (JEOL, Japan) were used at the UNIST (Ulsan National Institute of Science and Technology) Central Research Facilities Center (UCRF) of the UNIST. Focused ion beam (FEI, USA) milling was used to prepare the TEM specimens. Mo grids were used for the HRTEM–EDS analysis of Pd–Cu NCs. The average atomic percentage of Pd:Cu was 93.1:6.9 ( Supplementary Fig. S11 ). The average atomic percentage of Pd:Au was 5.2:1 according to a quantitative analysis of Pd–Au NPs by FESEM–EDS ( Supplementary Fig. S12 ). The average atomic percentage of Pd:Co in the Pd–Co NPs was 94.7:5.3 according to FESEM–EDS ( Supplementary Fig. S13 ). How to cite this article: Lee, J.-Y. et al. Hydrogen-atom-mediated electrochemistry. Nat. Commun. 4:2766 doi: 10.1038/ncomms3766 (2013).